Inhibition of CRISPR-Cas9 ribonucleoprotein complex assembly by anti-CRISPR AcrIIC2 CRISPR-Cas adaptive immune systems function to protect bacteria from invasion by foreign genetic elements. The CRISPR-Cas9 system has been widely adopted as a powerful genome-editing tool, and phage-encoded inhibitors, known as anti-CRISPRs, offer a means of regulating its activity. Here, we report the crystal structures of anti-CRISPR protein AcrIIC2 Nme alone and in complex with Nme1Cas9. We demonstrate that AcrIIC2 Nme inhibits Cas9 through interactions with the positively charged bridge helix, thereby preventing sgRNA loading. In vivo phage plaque assays and in vitro DNA cleavage assays show that AcrIIC2 Nme mediates its activity through a large electronegative surface. This work shows that anti-CRISPR activity can be mediated through the inhibition of Cas9 complex assembly. CRISPR-Cas systems provide adaptive immunity that protects bacteria and archaea against invasion by phages, plasmids, and other foreign genetic elements [1] , [2] , [3] . When a bacterial cell is invaded by a phage, the CRISPR-Cas system acquires a short segment of the phage genome and integrates it into the CRISPR locus where it can serve as a template for the production of mature CRISPR RNA (crRNA) molecules. These crRNAs form a complex with either a single protein effector or a multi-subunit effector complex that targets and degrades invading nucleic acids in a sequence-specific manner. CRISPR-Cas systems are divided into two classes, which can be further subdivided into six types and 33 subtypes, including their variants [4] . Class 1 systems (types I, III, and IV) form multi-subunit effector complexes, while Class 2 systems (types II, V, and VI) use a single protein to target invading genetic elements [5] . The type II protein, Cas9, has been widely adapted as a molecular tool for genome editing purposes. In response to the evolutionary pressures posed by active CRISPR-Cas systems, phages have evolved protein inhibitors of these systems. The first described anti-CRISPR proteins were active against the type I-E and I-F systems in Pseudomonas aeruginosa [6] , [7] , [8] . Subsequently, anti-CRISPR proteins were identified against type II-C [9] , [10] , type II-A [11] , [12] , [13] , type I-D [14] , type I-C [15] , and type V-A [15] , [16] CRISPR-Cas systems. The protein sequences of these anti-CRISPRs display high sequence diversity and the mechanisms by which they function also vary widely. Within the type I systems, anti-CRISPRs AcrIF1, AcrIF2, and AcrIF10 have been shown to interact directly with the Cascade complex and block DNA binding [17] , [18] , [19] , [20] , [21] . AcrIF3 interacts with the Cas3 nuclease and prevents its recruitment to the DNA-bound Cascade complex [22] , while AcrIF10 acts as a DNA mimic, binding to the basic residues that are critical for DNA binding. The mechanisms of activity of the type II anti-CRISPRs have proven to be similarly varied. Type II-C anti-CRISPR AcrIIC1 was shown to bind directly to the Cas9 HNH domain and prevent cleavage of the target DNA strand, while AcrIIC3 was shown to induce Cas9 dimerization and thereby inhibit DNA binding activity [23] . AcrIIA4 and AcrIIA2, which inhibit type II-A Cas9 proteins, were shown to occupy the PAM-interacting site, interacting with the RuvC, CTD, and TOPO domains of SpyCas9, and inhibiting the nuclease activity of SpyCas9 through multiple mechanisms [24] . Thus, previously characterized anti-CRISPRs function either through inhibition of nuclease activity or by blocking target DNA binding. As Cas9 is a large multi-functional protein that mediates its activities through multiple domains, it provides a variety of surfaces that could potentially be targeted by anti-CRISPRs. Cas9 is composed of two lobes, the α-helical recognition (REC) lobe and the nuclease (NUC) lobe. The NUC lobe contains the HNH and RuvC endonuclease domains that are required for DNA cleavage activity, and the more variable PAM-interacting domain (PID). The two lobes are connected by the arginine-rich bridge helix. The PID is largely disordered in the apo-Cas9 structure, which prevents target DNA recognition in the absence of guide RNA. The transition of Cas9 to its active conformation requires binding of a guide RNA molecule [25] , [26] . This results in substantial structural rearrangements, with the most prominent conformational changes taking place in the REC lobe [27] . Binding to both target DNA and guide RNA are thought to be key regulators of Cas9 enzyme function [26] . In this work, we investigate the mechanism of activity of anti-CRISPR protein AcrIIC2 Nme . This 123-residue protein was previously shown to inhibit the activity of Neisseria meningitidis CRISPR-Cas9 in vivo and in vitro [9] , [23] . We show that AcrIIC2 Nme functions by inhibiting loading of the guide RNA molecule, thereby preventing formation of the active CRISPR-Cas9 surveillance complex. As previously characterized mechanisms of anti-CRISPR activity all target fully assembled CRISPR-Cas complexes, AcrIIC2 Nme provides a unique mechanism for anti-CRISPR activity. AcrIIC2 Nme binds to the bridge helix We previously showed that anti-CRISPR protein AcrIIC2 Nme was able to robustly inhibit the cleavage activity of the N. meningitidis type II-C CRISPR-Cas9 protein [9] , [23] . As other anti-CRISPRs have been shown to have activity against multiple Cas9 orthologues [23] , we investigated the range of activity of AcrIIC2 Nme using an in vivo phage-targeting assay (Fig. 1a ). In this assay, the Cas9 protein is expressed from a plasmid in Escherichia coli together with an sgRNA that targets E. coli phage Mu. This CRISPR targeting prevents phage Mu from forming plaques. In the presence of a functional anti-CRISPR protein, phage Mu is able to successfully infect the bacterial cell, leading to plaque formation. We determined that AcrIIC2 Nme was able to fully inhibit the activity of its cognate type II-C Cas9 protein from N. meningitidis (Nme1Cas9), as well as a homolog from Haemophilus parainfluenzae (HpaCas9) that shares 65% sequence identity [10] . By contrast, AcrIIC2 Nme showed very poor inhibitory activity against the type II-C Cas9 proteins from Geobacillus stearothermophilus (GeoCas9) and Campylobacter jejuni (CjeCas9), which share only 38% and 31% sequence identity with Nme1Cas9. These results are consistent with our previous work that showed AcrIIC2 Nme inhibits Nme1Cas9 and HpaCas9, but not more distantly related Cas9 proteins in vitro [10] , [23] . Fig. 1 AcrIIC2 Nme inhibits Cas9 activity through an interaction with the bridge helix. a Plaquing of E. coli phage Mu targeted by type II-C Cas9 proteins (Nme1Cas9, HpaCas9, GeoCas9, CjeCas9) in the presence of AcrIIC2 Nme , a type II-C anti-CRISPR with broad activity (AcrIIC1 Nme ) and a type I anti-CRISPR (AcrIE2). The sequence identity of the Cas9 proteins as compared to Nme1Cas9 is noted to the right of the figure. b Untagged anti-CRISPR was co-purified with 6x-His-tagged full-length HpaCas9, or domains thereof ( c ) using Ni-NTA affinity chromatography and the bound proteins were analyzed by SDS-PAGE and visualized using Coomassie staining. c Schematics of HpaCas9 truncations used to identify the domain with which AcrIIC2 Nme interacts. The bridge helix is denoted in dark gray, and the three sequence regions that comprise the RuvC domain are denoted as I, II, and III Full size image To gain insight into how AcrIIC2 Nme inhibits Cas9 activity, we set out to identify the domain with which it interacts. Full-length Nme1Cas9 was susceptible to degradation in vivo and many of its isolated domains were insoluble. Thus, we used the closely related HpaCas9 for these studies because the holoenzyme and isolated domains were considerably more stable than Nme1Cas9. We co-expressed untagged AcrIIC2 Nme with 6-His-tagged HpaCas9 in E. coli and purified the resulting complex using Ni-affinity chromatography. AcrIIC2 Nme co-purified with Cas9, showing a specific interaction between the two proteins (Fig. 1b ). We next tested for interactions with isolated Cas9 domains, including the HNH domain, the guide RNA recognition (REC) lobe, and the PID (Fig. 1c ). We found that AcrIIC2 Nme co-eluted from the Ni-NTA column with the REC lobe (Fig. 1b ). To further delineate the region of the REC lobe with which AcrIIC2 Nme interacts, we created a construct lacking the N-terminal arginine-rich bridge helix (REC-ΔBH). AcrIIC2 Nme was unable to stably interact with this domain. To determine if the bridge helix alone was sufficient for AcrIIC2 Nme binding to Cas9, we created a deletion mutant of Cas9 that maintained the bridge helix but lacked the REC1 and REC2 domains (ΔREC1/2). AcrIIC2 Nme still bound to this protein. Consistent with the bridge helix interaction, AcrIIC2 Nme did not bind to the isolated HNH or PID and was able to bind to Cas9 in their absence (Fig. 1b ). These results indicate that the bridge helix is the primary binding site for AcrIIC2 Nme . The interaction of AcrIIC2 Nme inhibits sgRNA binding The Cas9 REC lobe mediates sgRNA binding [28] . To determine the effects of AcrIIC2 Nme on sgRNA binding, we co-expressed it in E. coli with His-tagged Nme1Cas9 and sgRNA and purified the resulting complex using affinity chromatography. AcrIIC2 Nme co-purified with Nme1Cas9, but no sgRNA was bound to the complex (Fig. 2a ). By contrast, when Nme1Cas9-sgRNA was co-expressed with a type I-E anti-CRISPR protein, which does not inhibit Cas9, the sgRNA co-purified with Nme1Cas9 (Fig. 2a ). Thus, the interaction of AcrIIC2 Nme with Nme1Cas9 appears to block sgRNA binding to Nme1Cas9. In addition, we observed increased proteolysis of Nme1Cas9 when it was co-expressed with AcrIIC2 Nme (Fig. 2a ). Previous work has shown that the Cas9 apo protein binding to guide RNA results in conformational changes that render the protein more resistant to proteolysis [26] , [29] , [30] . These conformational changes are required to form the active complex for target DNA cleavage. The increased sensitivity of Cas9 to cellular proteases in the presence of AcrIIC2 Nme is consistent with its role in blocking sgRNA binding. To further probe whether the binding of AcrIIC2 Nme affects the assembly of the Nme1Cas9-sgRNA surveillance complex, we performed limited α-chymotrypsin proteolysis. Both apo-Nme1Cas9 and AcrIIC2 Nme -bound Nme1Cas9 were sensitive to α-chymotrypsin, and they exhibited similar digestion patterns (Supplementary Fig. 1A ). By contrast, Nme1Cas9 bound to sgRNA or sgRNA/target DNA showed increased resistance to proteolysis (Supplementary Fig. 1B ). When apo-Nme1Cas9 was pre-incubated with AcrIIC2 Nme and then sgRNA or sgRNA/target DNA was added, the digestion patterns were similar to those observed for apo-Nme1Cas9, indicating that prior interaction with AcrIIC2 Nme blocked sgRNA binding (Supplementary Fig. 1C ). Finally, size exclusion chromatography was used to verify that AcrIIC2 Nme forms a stable complex with Nme1Cas9 but is unable to interact with sgRNA-bound Nme1Cas9 complex (Fig. 2b ). Taken together, these results imply that AcrIIC2 Nme inhibits Nme1Cas9 by disrupting the assembly of the Nme1Cas9-sgRNA complex. Fig. 2 AcrIIC2 Nme inhibits sgRNA binding. a Purification of His-tagged Nme1Cas9 + sgRNA co-expressed with AcrIIC2 Nme or a type I anti-CRISPR protein (AcrIE2) using Ni-NTA chromatography. Analysis of the resulting elutions included SDS-PAGE followed by Coomassie staining (upper panel) and denaturing polyacrylamide/urea gel followed by SYBR Gold staining (lower panel). b Gel filtration chromatography shows that AcrIIC2 Nme interacts with sgRNA-free Nme1Cas9 (upper panel), but fails to bind to the Nme1Cas9-sgRNA complex (lower panel). The Nme1Cas9-sgRNA-AcrIIC2 Nme and Nme1Cas9-AcrIIC2 Nme -sgRNA samples were reconstituted by incubation of purified Nme1Cas9, sgRNA, and AcrIIC2 Nme at a molar ratio of 1:1.3:4 on ice. Each component was added in the order listed, with an intermittent incubation of 30 min before adding the next component. All samples were fractionated on a Superdex 200 increase 10/300, and fractions between 11 and 13 mL were analyzed on SDS-PAGE. c Radiolabeled RNAs were incubated with increasing amounts of Nme1Cas9 in the absence (gray) or presence (purple) of AcrIIC2 Nme , and the fraction of protein-bound RNA was determined by nitrocellulose filter binding. Source data are provided as a Source Data file. d DNA cleavage assays with Nme1Cas9 and AcrIIC2 Nme . The components and order of addition are noted above each lane. The AcrIIC2 Nme mutants were mixed with Nme1Cas9 before adding the sgRNA Full size image To validate our observation that AcrIIC2 Nme inhibits the loading of sgRNA onto Nme1Cas9, we tested the ability of Nme1Cas9 to bind sgRNA in the absence and presence of AcrIIC2 Nme using a filter-binding assay. This revealed that addition of AcrIIC2 Nme at a four-fold molar ratio decreased the affinity of binding of sgRNA to Nme1Cas9 (Fig. 2c ). Using isothermal calorimetry (ITC) we calculated binding affinities for AcrIIC2 Nme and sgRNA to apo-Nme1Cas9. We determined that AcrIIC2 Nme bound with a K d of 200 nM, while the affinity of the sgRNA was ten times greater ( K d = 23 nM; Supplementary Fig. 2 ). When we added a two-fold molar excess of AcrIIC2 Nme to Nme1Cas9 before sgRNA addition, we found that the affinity of sgRNA binding decreased to 76 nM. When a 20-fold molar excess of AcrIIC2 Nme was added before sgRNA, the affinity of sgRNA binding decreased further, to 3.2 μM. Gel filtration chromatography was also used to analyze the equilibrium complexes formed under these reaction conditions. We found that some Nme1Cas9-sgRNA complex was present in the presence of a two-fold excess of AcrIIC2 Nme , but not in the presence of 10-fold excess AcrIIC2 Nme (Supplementary Fig. 3A ). These results indicate that AcrIIC2 Nme competes with sgRNA for the binding site on Nme1Cas9 and prevents formation of the active surveillance complex. We next used in vitro competition assays to evaluate the competition between AcrIIC2 Nme and sgRNA for the binding site on Nme1Cas9. When sgRNA was mixed with Nme1Cas9, and then AcrIIC2 Nme was added to this pre-formed complex, there was no inhibition of DNA cleavage (Fig. 2d ). When AcrIIC2 Nme was pre-bound to Nme1Cas9 at a ratio of 2:1 and then an equal amount of sgRNA was added, we found complete inhibition of DNA cleavage in vitro (Fig. 2d , Supplementary Fig. 3B ). However, when sgRNA and AcrIIC2 Nme were added simultaneously, a two-fold excess of AcrIIC2 Nme did not appreciably inhibit Nme1Cas9 activity (Supplementary Fig. 3B ). In fact greater than 10-fold excess of anti-CRISPR was required to block DNA cleavage activity under these conditions (Supplementary Fig. 3B ). Collectively, these data show that the anti-CRISPR and sgRNA directly compete for the same binding site. AcrIIC2 Nme is able to interact with Nme1Cas9 and block its activity through disruption of sgRNA binding, however, it does not efficiently inhibit the activity of the pre-formed surveillance complex due to its weaker binding interaction with Nme1Cas9. AcrIIC2 Nme has an electronegative functional surface To better understand the precise mechanism by which AcrIIC2 Nme inhibits Cas9 activity, we determined its crystal structure to a resolution of 2.5 Å using single-wavelength anomalous diffraction (SAD). 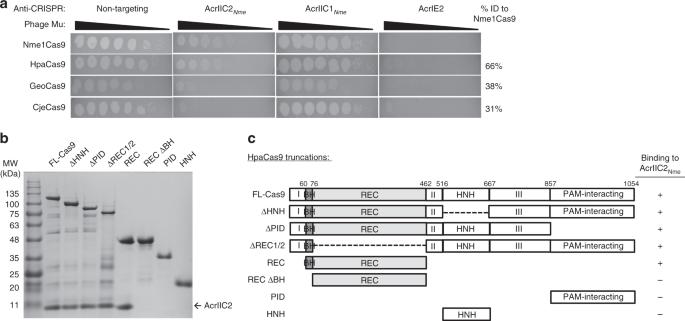Fig. 1 AcrIIC2Nmeinhibits Cas9 activity through an interaction with the bridge helix.aPlaquing ofE. coliphage Mu targeted by type II-C Cas9 proteins (Nme1Cas9, HpaCas9, GeoCas9, CjeCas9) in the presence of AcrIIC2Nme, a type II-C anti-CRISPR with broad activity (AcrIIC1Nme) and a type I anti-CRISPR (AcrIE2). The sequence identity of the Cas9 proteins as compared to Nme1Cas9 is noted to the right of the figure.bUntagged anti-CRISPR was co-purified with 6x-His-tagged full-length HpaCas9, or domains thereof (c) using Ni-NTA affinity chromatography and the bound proteins were analyzed by SDS-PAGE and visualized using Coomassie staining.cSchematics of HpaCas9 truncations used to identify the domain with which AcrIIC2Nmeinteracts. The bridge helix is denoted in dark gray, and the three sequence regions that comprise the RuvC domain are denoted as I, II, and III All X-ray data collection and refinement statistics are summarized in Table 1 . To date, the structures of 11 anti-CRISPR proteins have been determined [for review see ref. [31] ]. These anti-CRISPR families share no sequence identity and all display very different protein structures. Consistent with these previous observations, AcrIIC2 Nme shares no sequence or structural similarity with previously characterized anti-CRISPR proteins. A DALI search [32] of the Protein Data Bank also did not reveal any significant similarity to any previously determined structure. The protein architecture of AcrIIC2 Nme consists of a six-stranded β-sheet composed of two anti-parallel β-strands followed by a Greek key motif, all wrapped around a 20-residue α-helix (Fig. 3a ). Table 1 Data collection and refinement statistics Full size table Fig. 3 AcrIIC2 Nme functions as a homodimer. a The crystal structure of AcrIIC2 Nme solved by Se-SAD reveals a dimeric protein containing both α-helical and β-strand structural elements. Monomers are colored in violet and deep salmon, and the N- and C-termini are noted. b Cartoon representation of AcrIIC2-Nme1Cas9 complex. c Surface representation of AcrIIC2-Nme1Cas9 complex. d Electrostatic surface potential of AcrIIC2-Nme1Cas9 complex. e , f Interactions between the bridge helix and AcrIIC2 Nme . The bridge helix is shown in cyan. AcrIIC2.1 and AcrIIC2.2 are shown in violet and deep salmon, respectively Full size image We also solved the crystal structure of AcrIIC2 Nme in complex with Nme1Cas9 to a resolution of 2.6 Å. We found that AcrIIC2 Nme bound to Nme1Cas9 in the same dimeric form as observed in the unbound state (Fig. 3b, c ). Unexpectedly, only residues 16–77 of Nme1Cas9, corresponding to the bridge helix region and a partial fragment I of the RuvC domain, were observed in the complex (Supplementary Fig. 4A ). Analysis of the AcrIIC2-Nme1Cas9 crystal by SDS-PAGE revealed that the rest of Nme1Cas9 was digested during crystallization. To confirm this finding, we treated the AcrIIC2-Nme1Cas9 complex with α-chymotrypsin protease, and then crystalized the digested complex. We solved this structure to a resolution of 2.3 Å and found that it was similar to the structure discussed above (Supplementary Fig. 4B and C ). This further confirms that the bridge helix is the primary target for AcrIIC2 Nme activity. We next analyzed interactions between AcrIIC2 Nme and Nme1Cas9. As shown in Fig. 3d , the AcrIIC2 Nme monomers form a dimer with a negatively charged surface on one side into which the arginine-rich bridge helix nestles. Four residues from each of the AcrIIC2 Nme monomers, E17, E24, D108, and N112, make interactions with the bridge helix (Fig. 3e, f ). In AcrIIC2.1, the side-chain of E17 hydrogen bonds with Nme1Cas9 residues R69 and R73, E24 interacts with residues R73 and R74, while D108 and N112 form hydrogen bonds with the side-chain of R74. Similarly, the side-chains of E24, D108, E17, and N112 of AcrIIC2.2 interact with Nme1Cas9 residues R62, R66, R69, and R70. To determine if the interactions between AcrIIC2 Nme and the bridge helix of Nme1Cas9 are required and sufficient for anti-CRISPR inhibitory activity, we mutated 19 residues distributed widely across the surface of AcrIIC2 Nme (Fig. 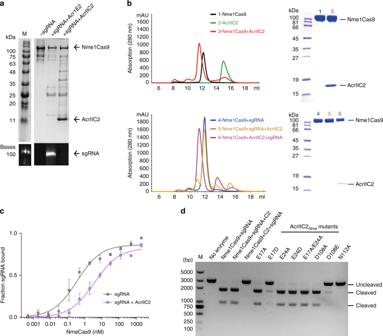Fig. 2 AcrIIC2Nmeinhibits sgRNA binding.aPurification of His-tagged Nme1Cas9 + sgRNA co-expressed with AcrIIC2Nmeor a type I anti-CRISPR protein (AcrIE2) using Ni-NTA chromatography. Analysis of the resulting elutions included SDS-PAGE followed by Coomassie staining (upper panel) and denaturing polyacrylamide/urea gel followed by SYBR Gold staining (lower panel).bGel filtration chromatography shows that AcrIIC2Nmeinteracts with sgRNA-free Nme1Cas9 (upper panel), but fails to bind to the Nme1Cas9-sgRNA complex (lower panel). The Nme1Cas9-sgRNA-AcrIIC2Nmeand Nme1Cas9-AcrIIC2Nme-sgRNA samples were reconstituted by incubation of purified Nme1Cas9, sgRNA, and AcrIIC2Nmeat a molar ratio of 1:1.3:4 on ice. Each component was added in the order listed, with an intermittent incubation of 30 min before adding the next component. All samples were fractionated on a Superdex 200 increase 10/300, and fractions between 11 and 13 mL were analyzed on SDS-PAGE.cRadiolabeled RNAs were incubated with increasing amounts of Nme1Cas9 in the absence (gray) or presence (purple) of AcrIIC2Nme, and the fraction of protein-bound RNA was determined by nitrocellulose filter binding. Source data are provided as aSource Datafile.dDNA cleavage assays with Nme1Cas9 and AcrIIC2Nme. The components and order of addition are noted above each lane. The AcrIIC2Nmemutants were mixed with Nme1Cas9 before adding the sgRNA 4a and Table 2 ). We also created a mutant lacking the final 12 amino acids (Δ112–123), which were not resolved in one of the apo crystal structures. The anti-CRISPR activity of each mutant was tested using the in vivo phage-targeting assay, in which expression of wild type AcrIIC2 Nme inactivates Nme1Cas9 and allows phage Mu to plaque. Mutation of three of the four amino acids that make direct contacts with the bridge helix (E17A, E24A, D108A) displayed a complete lack of anti-CRISPR activity in vivo (Fig. 4b and Table 2 ) while the other mutants showed changes in activity of less than 10-fold. Deletion of residue N112 (Δ112–123 mutant) did not affect activity. In vitro DNA cleavage assays further verified these results. Substitution of E17, E24, and D108 with Ala severely inhibited the activity of AcrIIC2 Nme , as did the variant E24D (Fig. 2d ). By contrast, mutants that maintained the negative charge at two of these positions (E17D and D108E) had similar levels of inhibition to that of wild type AcrIIC2 Nme . Circular dichroism spectroscopy of the three mutants with abrogated in vivo activity revealed spectra similar to the wild type protein (Fig. 4c ), showing that the lack of activity was not due to a folding defect. 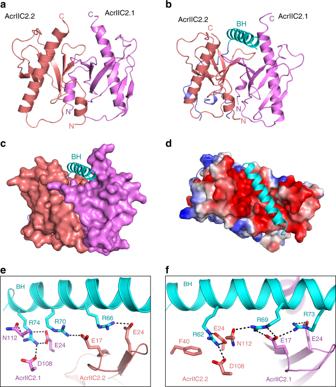Fig. 3 AcrIIC2Nmefunctions as a homodimer.aThe crystal structure of AcrIIC2Nmesolved by Se-SAD reveals a dimeric protein containing both α-helical and β-strand structural elements. Monomers are colored in violet and deep salmon, and the N- and C-termini are noted.bCartoon representation of AcrIIC2-Nme1Cas9 complex.cSurface representation of AcrIIC2-Nme1Cas9 complex.dElectrostatic surface potential of AcrIIC2-Nme1Cas9 complex.e,fInteractions between the bridge helix and AcrIIC2Nme. The bridge helix is shown in cyan. AcrIIC2.1 and AcrIIC2.2 are shown in violet and deep salmon, respectively In addition, cooperative thermal denaturation curves and melting temperatures similar to the wild type protein (Table 3 ) indicated that these mutants maintained stable, folded structures. We conclude that the negatively charged surface of AcrIIC2 Nme and the positively charged Nme1Cas9 bridge helix comprise a critical interaction interface that is required for anti-CRISPR activity. Fig. 4 AcrIIC2 Nme activity is mediated through a large electronegative surface. a AcrIIC2 Nme surface-exposed residues targeted for site-directed mutagenesis are shown on the surface of the protein. The side chain positions at which amino acid substitutions did not affect activity are shown in gray, while the three residues that showed the large decrease in activity when substituted are shown in red. b Representative results of the in vivo phage plaque assay. Serial dilutions of phage Mu plated on E. coli reveal that E17A, E24A, and D108A mutants have lost the ability to inhibit CRISPR-Cas9. c Representative circular dichroism spectroscopy scans of wild type anti-CRISPR (red) and three inactive mutants (E17A, blue; E24A, green; D108A, purple) show that the inactive mutants maintain their secondary structure. d Co-purification of AcrIIC2 Nme mutants with 6x-His-tagged Nme1Cas9 reveals decreased binding of the inactive anti-CRISPRs to Nme1Cas9, and corresponding increase in the amount of Cas9-bound sgRNA. e In vitro DNA cleavage assays with wild type Nme1Cas9 and the site-directed mutants in the bridge helix domain in the presence and absence of AcrIIC2 Nme . f Sequence alignment of the bridge helix of Nme1Cas9 and SpyCas9. The residue numbers of Nme1Cas9 are shown above the sequence. The amino acids that are identical in both Nme1Cas9 and SpyCas9 are shown with yellow background. The Nme1Cas9 amino acids that interact with AcrIIC2 Nme are shown in red. Residues T62 and T73 of SpyCas9 are highlighted by blue stars. g DNA cleavage assay with the wild type or mutant SpyCas9 either in the presence or absence of AcrIIC2 Nme to test whether AcrIIC2 Nme protein inhibits the activity of SpyCas9 mutants Full size image Table 2 In vivo phage plaquing assays Full size table Table 3 Thermal stability values ( T m ) derived by circular dichroism spectroscopy Full size table To further validate this functional surface, we assayed the ability of non-functional AcrIIC2 Nme mutants to inhibit sgRNA binding. We co-expressed His-tagged Nme1Cas9 with its sgRNA from a plasmid in E. coli and introduced a second plasmid that expressed either wild type AcrIIC2 Nme , one of the inactive mutants, or a type I-E anti-CRISPR protein. Using nickel affinity chromatography we purified Nme1Cas9 and the associated sgRNA and anti-CRISPR proteins. In the absence of anti-CRISPR or in the presence of a control anti-CRISPR that targets the type I-E system, sgRNA co-purified with Nme1Cas9 (Fig. 4d ). In the presence of wild type AcrIIC2 Nme , no sgRNA co-purified, confirming the ability of this anti-CRISPR to block sgRNA binding in vivo. The inactive mutants showed varying levels of binding to Nme1Cas9, resulting in varying levels of inhibition of sgRNA binding (Fig. 4d ). E17A was severely compromised, while E24A showed some inhibition of sgRNA binding, but not as strong as the wild type anti-CRISPR protein. Interestingly, both E24A and D108A maintained the ability to bind to Nme1Cas9, but were outcompeted by the sgRNA when it was added to the pre-formed AcrIIC2 Nme -Nme1Cas9 complex (Supplementary Fig. 5A,B ). Moreover, a double mutant, E17A/E24A, was completely outcompeted by the sgRNA (Supplementary Fig. 5C ). These results further confirm that the acidic residues of AcrIIC2 Nme are crucial for the inhibition of Nme1Cas9. We next examined residues in the Nme1Cas9 bridge helix that interact with AcrIIC2 Nme in the crystal structure. We first targeted position R62 and showed that substitution with Ala decreased inhibition of Nme1Cas9 by wild type AcrIIC2 Nme . By contrast, substitution with Lys, which maintains the charge interaction with residue E24 in AcrIIC2 Nme , allowed the anti-CRISPR to retain its inhibitory activity (Fig. 4e ). These data suggest that the interaction between R62 of Nme1Cas9 and E24 of AcrIIC2.2 is crucial for inhibition. 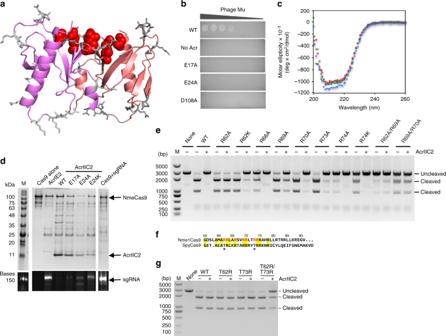Fig. 4 AcrIIC2Nmeactivity is mediated through a large electronegative surface.aAcrIIC2Nmesurface-exposed residues targeted for site-directed mutagenesis are shown on the surface of the protein. The side chain positions at which amino acid substitutions did not affect activity are shown in gray, while the three residues that showed the large decrease in activity when substituted are shown in red.bRepresentative results of the in vivo phage plaque assay. Serial dilutions of phage Mu plated onE. colireveal that E17A, E24A, and D108A mutants have lost the ability to inhibit CRISPR-Cas9.cRepresentative circular dichroism spectroscopy scans of wild type anti-CRISPR (red) and three inactive mutants (E17A, blue; E24A, green; D108A, purple) show that the inactive mutants maintain their secondary structure.dCo-purification of AcrIIC2Nmemutants with 6x-His-tagged Nme1Cas9 reveals decreased binding of the inactive anti-CRISPRs to Nme1Cas9, and corresponding increase in the amount of Cas9-bound sgRNA.eIn vitro DNA cleavage assays with wild type Nme1Cas9 and the site-directed mutants in the bridge helix domain in the presence and absence of AcrIIC2Nme.fSequence alignment of the bridge helix of Nme1Cas9 and SpyCas9. The residue numbers of Nme1Cas9 are shown above the sequence. The amino acids that are identical in both Nme1Cas9 and SpyCas9 are shown with yellow background. The Nme1Cas9 amino acids that interact with AcrIIC2Nmeare shown in red. Residues T62 and T73 of SpyCas9 are highlighted by blue stars.gDNA cleavage assay with the wild type or mutant SpyCas9 either in the presence or absence of AcrIIC2Nmeto test whether AcrIIC2Nmeprotein inhibits the activity of SpyCas9 mutants 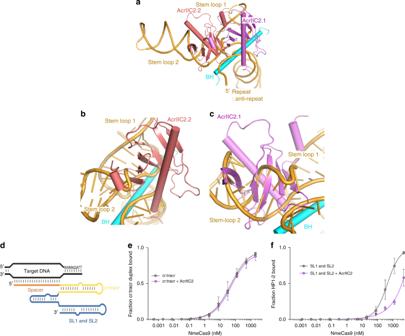Fig. 5 AcrIIC2Nmeblocks binding of the sgRNA by occluding the binding sites for stem loops 1 and 2.aStructural comparison between AcrIIC2Nme-Nme1Cas9 and Nme1Cas9-sgRNA binary complex based on the superimposition of bridge helix regions. Monomer AcrIIC2.2 occupies the major groove where stem loop 2 should bind (b) while AcrIIC2.1 occupies the positions of stem loop 1 and the seed region (c).dSchematic sgRNA, indicating the repeat:anti-repeat (cr:tracr) and 3′ stem loop 1 and 2 (SL1, SL2). Radiolabeled sgRNA truncations were incubated with Nme1Cas9-AcrIIC2Nmecomplex and the fraction of protein-bound RNA was determined by nitrocellulose filter binding when only the cr:tracr (e) or 3′ stem loops 1 and 2 (f) were present. Source data are provided as aSource Datafile Similarly, mutation of position R69 in the bridge helix of Nme1Cas9, which slightly decreased DNA cleavage activity, dramatically reduced the inhibitory activity of AcrIIC2 Nme . Substitution of four other positively charged residues in the bridge helix (R66A, R70A, R73A, and R74A) had little effect on the inhibitory activity of AcrIIC2 Nme (Fig. 4e ). Together, these results indicate that the interactions between AcrIIC2 Nme and the bridge helix of Nme1Cas9 are essential for inhibition. To determine if the sequence of the bridge helix is sufficient for inhibition by AcrIIC2 Nme , we compared the amino acid sequence of Nme1Cas9, which is robustly inhibited by AcrIIC2 Nme , with SpyCas9, which is not inhibited. We identified two positions in the SpyCas9 bridge helix (T62 and T73) that are arginine residues in Nme1Cas9 (Fig. 4f ). We substituted these positions singly and in combination, and discovered that the in vitro DNA cleavage activity of the SpyCas9 double mutant was inhibited by AcrIIC2 Nme (Fig. 4g ). This further confirms the importance of the interaction between AcrIIC2 Nme and the bridge helix of Cas9. It also emphasizes a potential role for anti-CRISPRs in driving Cas9 evolution. AcrIIC2 Nme blocks binding of sgRNA stem loops 1 and 2 To further establish the impact of AcrIIC2 Nme binding on the assembly of Nme1Cas9 with sgRNA, we compared the structure of AcrIIC2 Nme bound to Nme1Cas9 with the Nme1Cas9-sgRNA binary complex by aligning the bridge helix regions. The structural superposition shows that two AcrIIC2 Nme monomers make major clashes with stem loops 1 and 2, and slightly overlap the seed region of the sgRNA (Fig. 5a ). Monomer AcrIIC2.2 occupies the major groove of stem loop 2, displacing the duplex formed by nucleotides 125–131:98–90 and the adjacent single-stranded region at the 5′-end of the sgRNA (Fig. 5b ). Monomer AcrIIC2.1 occupies the positions of nucleotides 84–87 and seed region from nucleotides 20–23 (Fig. 5c ). To confirm the importance of these interactions, we assessed the ability of truncated sgRNA constructs to bind Nme1Cas9 in the presence of AcrIIC2 Nme . We found that the 5′ cr:tracr duplex bound to Cas9 with equal affinities in the presence and absence of AcrIIC2 Nme (Fig. 5d, e ). By contrast, the interaction of the 3′ stem loops was inhibited in the presence of AcrIIC2 Nme (Fig. 5d, f ). These terminal stem loops have been shown to assist in stabilizing the sgRNA and supporting stable complex formation with the Cas9 protein [33] . These results confirm that AcrIIC2 Nme interferes with sgRNA binding through an interaction that blocks the binding site of the stem loops 1 and 2. Fig. 5 AcrIIC2 Nme blocks binding of the sgRNA by occluding the binding sites for stem loops 1 and 2. a Structural comparison between AcrIIC2 Nme -Nme1Cas9 and Nme1Cas9-sgRNA binary complex based on the superimposition of bridge helix regions. Monomer AcrIIC2.2 occupies the major groove where stem loop 2 should bind ( b ) while AcrIIC2.1 occupies the positions of stem loop 1 and the seed region ( c ). d Schematic sgRNA, indicating the repeat:anti-repeat (cr:tracr) and 3′ stem loop 1 and 2 (SL1, SL2). Radiolabeled sgRNA truncations were incubated with Nme1Cas9-AcrIIC2 Nme complex and the fraction of protein-bound RNA was determined by nitrocellulose filter binding when only the cr:tracr ( e ) or 3′ stem loops 1 and 2 ( f ) were present. Source data are provided as a Source Data file Full size image In this work, we investigated the mechanism of activity of anti-CRISPR protein AcrIIC2 Nme . We found that it blocks Cas9 binding to sgRNA, thereby inhibiting biogenesis of the surveillance complex. This interference is mediated through an interaction with the arginine-rich bridge helix, which connects the REC lobe to the NUC lobe. High-resolution studies of Cas9-sgRNA complexes with and without target DNA bound show that the bridge helix contacts the sgRNA, in particular the region that pairs with nucleotides nearest the PAM sequence in the target DNA [28] , [34] . The crystal structure of AcrIIC2 Nme revealed a highly negatively charged surface that binds to the positively charged bridge helix. Mutation of this electronegative surface decreases the affinity of AcrIIC2 Nme for Cas9, resulting in loss of anti-CRISPR activity. The bridge helix, which forms part of the endonuclease functional core, is a universal feature of Cas9 proteins [26] and thus provides a reliable target for inhibition by anti-CRISPR proteins. The targeting of a highly conserved domain by AcrIIC2 Nme is similar to that observed for AcrIIC1 Nme , which was shown to target the HNH endonuclease domain for inhibition [23] . Other previously characterized type I and type II anti-CRISPRs revealed two general mechanisms for blocking CRISPR-Cas activity. The most common mechanism observed to date is inhibition of DNA binding through a direct interaction with the CRISPR surveillance complex. The second mechanism is blocking DNA cleavage by inhibiting nuclease activity, either through interaction with a Cas9 endonuclease domain [23] or the Cas3 endonuclease protein in type I systems [17] , [22] . The mechanism of activity for AcrIIC2 Nme that we determined in this study, disruption of CRISPR-Cas surveillance complex assembly through an interaction with the bridge helix, is in agreement with the study recently published by Zhu et al. in which they examined mechanisms of inhibition for anti-CRISPR proteins AcrIIC2 Nme and AcrIIC3 Nme [35] . Like Zhu et al., we found that pre-binding sgRNA to Nme1Cas9 greatly reduced the ability of AcrIIC2 Nme to interact with the complex and inhibit DNA cleavage activity due to its much lower affinity for Cas9 as compared to the sgRNA. Using structural and biochemical analyses, we showed that AcrIIC2 Nme competes for the binding site of the sgRNA stem loops 1 and 2. In the natural CRISPR-Cas9 system, where the crRNA and tracrRNA are separate molecules instead of a single fused molecule as in the case of the sgRNA, AcrIIC2 Nme may compete more effectively with the tracrRNA for binding to Cas9. This might endow the anti-CRISPR with an increased ability to disrupt pre-formed surveillance complexes that are present in the cell when the phage infects. In addition to blocking the surveillance complex formation, the activity of AcrIIC2 Nme leaves the Cas9 protein trapped in its apo form, which is much more sensitive to the activity of cellular proteases than are the RNA- and DNA-bound forms. Thus, the introduction of this anti-CRISPR into a cell may lead to a decrease in the steady state levels of full-length Cas9 in the cell, providing an additional mechanism of anti-CRISPR activity. This activity of AcrIIC2 Nme may explain the differences we observed in the in vivo and in vitro assays. When AcrIIC2 Nme was co-expressed with Nme1Cas9 in vivo and the resulting complex was purified, no sgRNA was found to be associated with the complex (Fig. 2a ). This contrasted with in vitro experiments, in which a great excess of anti-CRISPR was required to inhibit sgRNA binding. AcrIIC2 Nme is robustly produced, soluble to high concentration, and resistant to bacterial proteases in E. coli . It accumulates to high levels in the cell that allow it to bind to Nme1Cas9 immediately as the Cas9 protein is being produced. The sgRNA, by contrast, is probably less stable in the cell due to the activity of cellular nucleases. For these reasons, the anti-CRISPR likely has a larger competitive advantage in vivo as compared with the purified in vitro system. The reduction of Nme1Cas9 steady-state levels in the presence of AcrIIC2 Nme was previously observed in mammalian cells [10] , and probably also contributes to the ability of AcrIIC2 Nme to efficiently inhibit genome editing in these cells. Other anti-CRISPRs that inhibit DNA binding or interfere with nuclease activity do not appear to share this type of two-pronged inhibitory mechanism. Additionally, the activity of AcrIIC2 Nme may also serve to inhibit spacer acquisition, which has been shown to be Cas9-dependent [36] , [37] . Inhibiting the formation of the active CRISPR-Cas9 surveillance complex intuitively seems that it would not provide an advantage to infecting phages, as they could not overcome the pre-assembled surveillance complexes. However, recent work has shown that multiple phages need to infect a cell in order to provide a critical mass of anti-CRISPR protein to overwhelm the CRISPR system [38] , [39] . Even anti-CRISPRs that inhibit fully formed surveillance complexes fail to inactivate the CRISPR-Cas system if the phage population numbers fall below a critical threshold. When phages infect but fail to replicate in cells with active CRISPR systems, they still produce small amounts of anti-CRISPR proteins that leave the bacterial cell in an immunocompromised state. Thus, AcrIIC2 Nme molecules produced by a phage that was ultimately destroyed by Cas9 could persist within the cell and inhibit CRISPR-Cas complexes assembled after the infection. This would, in turn, increase the likelihood of successful replication by the next infecting phage. The expression of AcrIIC2 Nme would also be an effective means for a prophage to keep the CRISPR system turned off once it integrated into the host genome. Thus, a phage encoding an anti-CRISPR that prevents assembly of the CRISPR-Cas9 complex may not be at an evolutionarily disadvantage to one that inhibits the pre-formed complex. The distinct mechanism of activity of AcrIIC2 Nme , inhibiting assembly of a CRISPR-Cas complex, further emphasizes the amazing diversity of inhibitors that phages have evolved to counteract the existential challenge posed by CRISPR-Cas systems. Plasmid construction Plasmids encoding the Cas9 proteins used in the in vivo phage-targeting assay were generated by Gibson assembly using primers listed in Supplementary Table 1 . The pGeoCas9-sgRNA plasmid [23] was used as the starting vector. GeoCas9 and its sgRNA were replaced with the variant Cas9 proteins and their corresponding sgRNAs (sequences listed in Supplementary Table 1 ). The sgRNAs were synthetized as part of gblock fragments (IDT) along with overhangs to clone using Gibson assembly. All fragments used in the assembly reactions were first amplified using Phusion High-Fidelity DNA Polymerase (Thermo Fisher Scientific). The reactions were prepared according to manufacturer’s recommendations and 2 μL of the assembly reaction solution were transformed in High Efficiency chemically competent E. coli cells (New England Biolabs). Clones were screened by restriction digestion and were sequence-verified. The Cas9-encoding plasmids were linearized with BsaI and ligated to DNA encoding crRNA targeting phage Mu, which were generated by annealing of two complementary oligonucleotides carrying overhanging BsaI ends. For expression and protein purification in E. coli , NcoI-HindIII DNA inserts encoding wild type and mutant AcrIIC2 Nme proteins from pCDF-1b plasmids were sub-cloned into a pHAT4 [40] expression plasmid such that the protein was expressed with an N-terminal 6-His tag. The boundaries for the HpaCas9 HNH, PID, and REC domains were determined by alignment with GeoCas9, whose domain boundaries were previously described [23] . These domains were cloned into expression plasmid pCDF-1b with a 6-His tag fused to their C-termini. Point mutations in acrIIC2 Nme were generated by site-directed mutagenesis. The desired nucleotide mutations were introduced in the middle of 40 bp complementary primers (Supplementary Table 1 ). Sixteen PCR cycles were performed using Phusion ® High-fidelity DNA polymerase (ThermoScientific), and the PCR products were treated with DpnI endonuclease. The sample was ethanol precipitated and transformed into DH5α cells. Plasmids were isolated and mutations confirmed by sequencing. Phage plaque assays Plasmids expressing the different Cas9 proteins containing a spacer targeting phage Mu were co-transformed in BB101 cells with a plasmid expressing wild type or mutant AcrIIC2 Nme . Cells containing both plasmids were subcultured in Lysogeny broth (LB) supplemented with chloramphenicol and streptomycin and grown for 2 h, at which point anti-CRISPR expression was induced with 0.01 mM IPTG for 3 h. 200 μL of cells were mixed with soft agar and top-plated on LB supplemented with both antibiotics and 200 ng mL −1 aTc, 0.2% arabinose, and 10 mM MgSO 4 . Serial dilutions of phage Mu were spotted on top and the plates were incubated overnight at 37 °C. Experiments were performed in triplicate, with representative replicates shown in the figure panels. Cas9-AcrIIC2 Nme pull-down experiments E. coli BL21 cells were co-transformed with 6-His-tagged HpaCas9 constructs in a pMCSG7 backbone [10] , and a pCDF-1b vector encoding untagged AcrIIC2 Nme . Cells were grown in Terrific Broth (TB) at 37 °C to an optical density of 0.8. Protein expression was induced by the addition of 1 mM IPTG for 18 h at 16 °C. Cells were lysed by sonication in binding buffer (50 mM Tris pH 7.5, 200 mM NaCl, 5% Glycerol, 20 mM Imidazole). Clarified lysates were bound to Ni-NTA agarose (Qiagen) for 30 min at 4 °C, washed with binding buffer supplemented with 30 mM imidazole and bound protein was eluted with buffer containing 300 mM imidazole. 6-His-tagged Nme1Cas9 + sgRNA [9] ribonucleoprotein with wild type or mutant AcrIIC2 Nme was purified using the same protocol. Complexes were analyzed by SDS-PAGE on a 15% Tris–Tricine gel and visualized by Coomassie staining. The amount of bound sgRNA was examined using a 12.5% polyacrylamide/urea gel and visualized by SYBR Gold (Thermo Fisher Scientific) staining. Experiments were performed in triplicate, with representative replicates shown in the figure panels. Filter binding assays Filter binding was performed as described previously [23] . Filter binding was conducted in 1× Binding Buffer (20 mM Tris, pH 7.5, 100 mM KCl, 5 mM MgCl 2 , 1 mM DTT, 5% (vol/vol) glycerol, 0.01% Igepal CA-630, 10 μg mL −1 yeast tRNA, and 10 μg mL −1 BSA). Nme1Cas9 was mixed with a 4× molar ratio of AcrIIC2 Nme at the maximum concentration in Binding Buffer and was diluted in 1× Binding Buffer. Less than 0.01 nM radiolabeled sgRNA or the indicated guide truncation was added and allowed to incubate for 30 min at 37 °C. During incubation Tufryn (Pall Corporation), Protran (Whatman), and Hybond-N+ (GE Healthcare) membranes were soaked in Binding Buffer omitting the detergent, yeast tRNA and BSA and arranged on a dot blot apparatus above two layers of Whatman paper. The complexing reactions were loaded onto the dot blot apparatus and vacuum was applied. The membranes were dried and visualized by phosphorimaging and quantified using ImageQuant. All experiments were carried out in triplicate, with averaged values shown in the figure panels. Data were fit to a binding isotherm using Prism (GraphPad Software), and K d values of 0.24 ± 0.14 nM for sgRNA alone, and 2.2 ± 1.3 nM in the presence of AcrIIC2 Nme were determined. The sgRNA sequences for the truncation binding experiments are as follows: Full length sgRNA—GGTCTGTAAGCGGATGCCATATGGTTGTAGCTCCCTTTCTCGAAAGAGAACCGTTGCTACAATAAGGCCGTCTGAAAAGATGTGCCGCAACGCTCTGCCCCTTAAAGCTTCTGCTTTAACGGGCTT Repeat:anti-repeat—GGTTGTAGCTCCCTTTCTCGAAAGAGAACCGTTGCTACAATAA SL1 and SL2—GGCCGTCTGAAAAGATGTGCCGCAACGCTCTGCCCCTTAAAGCTTCTGCTTTAACGGGCTT Isothermal titration calorimetry Nme1Cas9, AcrIIC2 Nme , sgRNA and (Nme1Cas9-AcrIIC2 Nme ) complexes of 1:2, 1:10, and 1:20 molar ratios were extensively dialyzed against a buffer containing 300 mM NaCl, 20 mM Tris, pH 7.5. Titrations were performed using a MicroCal PEAQ-ITC system (Malvern Instruments) at 20 °C. To determine the affinity of binding for Nme1Cas9 and AcrIIC2 Nme , 100 μM AcrIIC2 Nme was titrated into 10 μM Nme1Cas9. To determine the affinities of sgRNA in the presence and absence of AcrIIC2 Nme , 90 μM Nme1Cas9 with or without AcrIIC2 Nme was titrated with 10 μM sgRNA. The resulting ITC curves were processed using Origin 7.0 software (OriginLab) using the “One Set of Sites” fitting model. Experiments were carried out in triplicate, with representative replicates shown in the figure panels. Competitive binding assays AcrIIC2 Nme , sgRNA, and Nme1Cas9 (molar ratios of 2:1:1, 3:1:1, or 10:1:1) were mixed together on ice and then centrifuged at 13,800× g at 4 °C for 10 min. The samples were loaded into a Superdex 200 Increase 10/300 (GE Healthcare) column for separation using gel filtration chromatography. The buffer used for gel filtration contained 300 mM NaCl, 20 mM Tris, pH 7.5. In vitro DNA cleavage assays The pUC19 target DNA plasmid (35 bp target DNA cloned into the pUC19 vector) was linearized by ScaI digestion before the cleavage reactions. In the presence or absence of AcrIIC2, the Cas9-sgRNA complex was incubated with 300 ng pUC19 target DNA in 10 μL reaction buffer containing 20 mM Tris–HCl pH 7.5, 100 mM KCl, 10 mM MgCl 2 , 1 mM DTT and 5% glycerol. All reactions were stopped by adding 1 μL 0.5 M EDTA and 1 μL 0.1 mg mL −1 Proteinase K for 30 min at room temperature. The reaction products were run on 1% agarose gels, and gels were stained with ethidium bromide for product detection. All experiments were carried out at least in triplicate, with representative replicates shown in the figure panels. Competitive cleavage assays For the competition cleavage assays, two incubation methods were employed to prepare the samples for DNA cleavage. First, Nme1Cas9 was incubated with AcrIIC2 Nme at molar ratios of 1:0, 1:2, 1:4, 1:10, 1:20, and 1:40 on ice for 15 min, 1.1 fold of sgRNA was added and the samples were incubated for an additional 15 min. Second, 1.1 fold of sgRNA was simultaneously mixed with AcrIIC2 Nme and Nme1Cas9 and incubated for 15 min on ice. The resulting enzyme complexes were incubated with 300 ng pUC19 target DNA in 10 μL reaction buffer (20 mM Tris–HCl pH 7.5, 100 mM KCl, 10 mM MgCl 2 , 1 mM DTT and 5% glycerol). The reactions were allowed to proceed at 37 °C for 10 min, and were stopped by the addition of 1 μL 0.5 M EDTA and 1 μL 0.1 mg mL −1 Proteinase K. The samples were incubated for 30 min at room temperature and the reaction products were run on 1% agarose gels and stained with ethidium bromide for product detection. All experiments were carried out at least in triplicate, with representative replicates shown in the figure panels. Purification of AcrIIC2 Nme The wild type and mutant AcrIIC2 Nme proteins were expressed in E. coli BL21 and purified as described previously [9] . Selenomethionine (Se-Met) labeled AcrIIC2 Nme was expressed using the methionine auxotrophic E. coli BL21(DE3) B834 strain cultured in M9 minimal media containing trace metals and supplemented with selenomethionine. Far-UV circular dichroism scans and thermal denaturation Purified wild type and mutant AcrIIC2 Nme proteins were dialyzed into 10 mM Tris pH 7.5, 0.2 mM EDTA, 250 mM KCl. The proteins were scanned on a Jasco J-810 CD Spectropolarimeter from 200 to 260 nm. Each scan was an average of five accumulations performed at 20 nm min −1 . For the thermal denaturation experiment, the proteins were heated at a rate of 1 °C min −1 from 20 to 90 °C, and the state of protein folding was assessed by absorbance at 218 nm. The assay was carried out with three biological replicates, and the standard deviation presented as the margin of error. Protein purification for Nme1Cas9-AcrIIC2 Nme co-crystals Full-length genes of AcrIIC2 Nme and Nme1Cas9 were purchased from Sangon Biotech, and cloned into an expression vector pET28a-Sumo with His6-Sumo tag at the N-terminus. Mutants were constructed using a site-directed mutagenesis kit. All proteins were overexpressed in E. coli Rosetta (DE3) (Novagen) cells and were induced with 0.1 mM isopropyl-1-thio-β-D-galactopyranoside (IPTG) at OD 600 = 0.6 for 12 h at 18 °C. Cells containing Nme1Cas9 were lysed by sonication in buffer containing in 20 mM Tris–HCl and 0.5 M NaCl, pH 7.5, at 4 °C. After centrifugation, the supernatant was purified by Ni Sepharose resin (GE Healthcare). Eluted Nme1Cas9 protein with His6-sumo-tag was digested with ubiquitin-like protein 1 (Ulp1) protease and dialyzed against 20 mM Tris–HCl, 0.3 M NaCl for 2 h at 4 °C to remove the His 6 -Sumo tag. Nme1Cas9 protein was further purified by Ni Sepharose column. Fractions were collected and purified on an SP column (GE Healthcare), eluting with buffer containing 20 mM Tris–HCl, pH 7.5, 1 M NaCl. Crystallization and structure determination of AcrIIC2 Nme Native and (Se-Met) Ni-NTA affinity-purified AcrIIC2 Nme proteins were further purified by size exclusion chromatography using a Superdex 75 column in buffer containing 20 mM Tris–HCl pH 7.5, 100 mM NaCl, 5 mM β-mercaptoethanol. Purified AcrIIC2 Nme was initially screened with 1:1 (protein:precipitant) ratio against the MCSG commercial suite and JCSG+ commercial screen using sitting drop vapor diffusion at 10 mg mL −1 . AcrIIC2 Nme crystals were observed in 0.1 M sodium citrate, 5% propanol, and 20% PEG 4000. The crystals were further optimized with a 1:1 ratio sitting drop at 20 °C in a precipitant condition composed of 0.1 M sodium citrate, 5% propanol and 18% PEG 4000 and 15% glycerol, yielding single crystals in space group P4 1 2 1 2. Crystallographic data was collected on crystals frozen at 105 K on the 08B1-1 beam line at Canadian Light Source (CLS). Diffraction data from a total of 360 images were collected at wavelengths of 0.9795 using 1° oscillations. Data were processed with XDS package to a resolution of 2.5 Å. A complete model for AcrIIC2 Nme was solved by Se-SAD with anomalous signal from Se atoms using Phenix AutoSol. The final model was generated after several rounds of model building and refinement using Coot and PHENIX refine programs using TLS, yielding a final R work / R free of 0.19/0.24. Structure determination of Nme1Cas9-AcrIIC2 Nme complex The Nme1Cas9-AcrIIC2 Nme complex was reconstituted on ice by incubating purified Nme1Cas9 and AcrIIC2 Nme at a molar ratio of 1:10. The resulting complex was purified by gel filtration chromatography, concentrated before crystallization to an absorbance of 280 nm to ~15, as measured by Nanodrop 2000, and then set for crystal screen. The Nme1Cas9-AcrIIC2-proteolysis complex was prepared by mixing Nme1Cas9 with AcrIIC2 Nme protein at a molar ratio of 1:10 on ice for 30 min. Subsequently, the sample was purified by gel filtration chromatography. Next, α-chymotrypsin was incubated with the complex at a mass ratio of 1:500 or 1:1000 before the sample was used for crystallization. The Nme1Cas9-AcrIIC2 complex was crystalized at 16 °C by hanging-drop vapor diffusion method. The Nme1Cas9-AcrIIC2 complex crystals were obtained by mixing 1 μL of complex solution and 1 μL of reservoir solution (0.1 M HEPES pH 7.5, 20% PEG 20,000, 0.01 M Phenol). Diffraction datasets were collected at beamline BL19U1 at Shanghai Synchrotron Radiation Facility and processed with XDS or HKL2000. The structure of the AcrIIC2-Nme1Cas9 complex was solved by molecular replacement with the AcrIIC2 dimer as the model. One Nme1Cas9-AcrIIC2 complex was identified in the asymmetric unit. The atomic model was built and refined using the programs Refmac and Phenix. Limited proteolysis of Nme1Cas9-AcrIIC2 Nme complex Limited α-chymotrypsin proteolysis assays were performed at 25 °C for different times (0, 10, 30, 60 min) using proteolysis buffer 20 mM Tris pH 7.5, 300 mM NaCl. The same amount (80 μg) of purified Nme1Cas9 was used to construct complex Nme1Cas9-sgRNA (1:1.1), Nme1Cas9-sgRNA-DNA (1:1.1:1.3), Nme1Cas9-AcrIIC2 (1:4), Nme1Cas9-AcrIIC2-sgRNA (1:4:1.1), Nme1Cas9-AcrIIC2-sgRNA-DNA (1:4:1.1:1.3). The reactions were stopped by adding 2× SDS loading buffer and quenched for 10 min at 70 °C. Samples were analyzed on a 15% SDS polyacrylamide gel with Tris–Glycine buffer. Reporting summary Further information on research design is available in the Nature Research Reporting Summary linked to this article.